Spatiotemporally controlled induction of autophagy-mediated lysosome turnover Lysosomes are the major degradative compartments within cells, harbouring a wide variety of hydrolytic enzymes within their lumen. Release of lysosomal hydrolases from lysosomes into the cell cytoplasm results in cell death. Here we report that damaged lysosomes undergo autophagic turnover. Using a light-induced lysosome impairing scheme that can be controlled spatially and temporally within a cell, we show that damaged lysosomes are selectively ubiquitinated, recruit autophagic proteins and are eventually incorporated into autolysosomes for degradation. We propose that autophagic removal of lysosomes, which we term lysophagy, is a surveillance mechanism that alleviates cells from the adverse effects of lysosomal damage. We envision our method to induce lysosomal damage will enable detailed molecular studies of the lysophagy pathway in the future. Lysosomes are ubiquitous cellular organelles responsible for the degradation of endocytosed entities as well as unwanted intracellular materials. The lysosomal degradative actions can be used to generate necessary nutrients from uptaken extracellular food sources, annihilate intruding pathogens and mobilize intracellularly stored materials through autophagy. Because of the large variety of hydrolytic enzymes contained within lysosomal lumens (to carry out the degradation of biomolecules), it was proposed more than 50 years ago by Nobel laureate Christian de Duve that release of lysosomal hydrolases from broken lysosomes into the cell cytoplasm would be detrimental to a cell [1] . Indeed, it is now established that treatment of cells with lysosomotropic agents that destabilize lysosomal membranes in detergent-like fashions cause the release of lysosomal hydrolases such as cathepsins into the cell cytoplasm, leading to apoptosis or necrosis [2] , [3] . This led us to hypothesize that the existence of lysosome-maintenance mechanisms will alleviate cells from potentially harmful effects of impaired lysosomes. One potential means to quality control lysosomes is through autophagy. Autophagy, the cellular pathway that targets cellular materials for degradation through the sequestration of cellular materials in double-layered membrane structures termed the phagophores, has already been implicated in the maintenance of cellular organelles such as mitochondria (mitophagy) and peroxisomes (pexophagy) [4] , [5] , [6] , [7] , [8] . One widely studied organelle-maintenance autophagic pathway is parkin-mediated mitophagy [8] . In this pathway, a loss of mitochondrial membrane potential is sensed by the PINK1/parkin machinery, leading to specific ubiquitination of outer-membrane proteins on damaged mitochondria [9] , [10] , [11] . This ubiquitin tag then allows the autophagic machinery and the autophagy adaptor protein p62 to specifically recognize and turnover a dysfunctional mitochondrion within the complex cellular environment [10] , [12] , [13] , [14] , [15] . In this study, we probe whether autophagy-based maintenance pathways also exist for lysosomes. Through a light-activation scheme, we observe that damaged lysosomes are selectively ubiquitinated, recruite autophagic proteins and are eventually incorporated into autolysosomes for degradation. These observations suggest that autophagy acts as one quality-control mechanism for lysosomes. Spatiotemporally controlled induction of lysosomal damage To probe whether lysosomes can be maintained by autophagy, we established a methodology that enables spatiotemporally controlled impairment of lysosomes within living cells. Lysosome impairment induced by small molecules, such as lysosomotropic agents, results in massive release of lysosomal hydrolases into the cell cytoplasm and triggers cell death responses [2] , [3] . These treatments inactivate lysosomes globally within a cell (all lysosomes can become targeted) and abrogate the ability of a cell to complete autophagic responses as that requires the presence of active lysosomes. This prompted us to seek alternative strategies in which limited lysosomal damage occurs, minimizing unwanted cell stress and preserving most lysosomes in a cell for possible autophagic clearance mechanisms. To achieve spatiotemporally controlled inactivation of lysosomes, we took advantage of a previously developed strategy for photochemical internalization, a process that facilitates gene delivery through efficient light-induced lysosome breakage [16] , [17] . In photochemical internalization, a robust photosensitizer is targeted onto lysosomal membranes. Light triggers reactive oxygen species formation at the lysosomal membrane, breaking lysosomes to allow gene delivery into the cell cytoplasm. We utilized disulfonated aluminium phthalocyanine (AlPcS 2a ), a robust photosensitizer that targets to lysosomes through endocytosis [18] . Through patterned 635 nm illumination [16] , AlPcS 2a containing lysosomes can be individually impaired with spatiotemporal precision ( Fig. 1a ). AlPcS 2a fluoresces in the far red, making it easy to combine with blue, green and red fluorescent protein constructs for live-cell imaging. 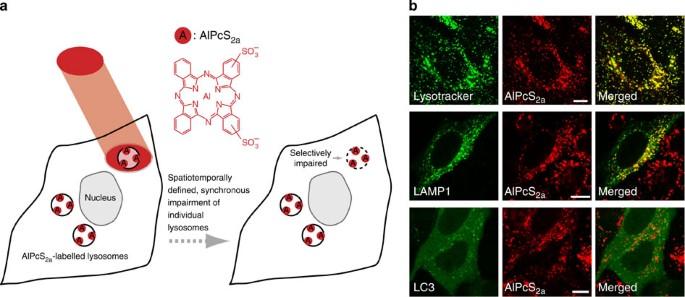Figure 1:Targeting AlPcS2aonto lysosomes for light-activated lysosomal damage. (a) Schematic for spatiotemporally controlled light-activated lysosomal damage. Illumination of individual lysosomes labelled with the robust photosensitizer AlPcS2aleads to light-activated damage. (b) AlPcS2acan be specifically targeted onto lysosomes. Using our staining procedure, AlPcS2asignals colocalized with Lysotracker Red (top panels) and lamp1-RFP (middle panels), but not with other cellular organelle markers such as EGFP-LC3B (bottom panels, marker for autophagic structures), in HeLa cells. Scale bars, 10 μm. Figure 1: Targeting AlPcS 2a onto lysosomes for light-activated lysosomal damage. ( a ) Schematic for spatiotemporally controlled light-activated lysosomal damage. Illumination of individual lysosomes labelled with the robust photosensitizer AlPcS 2a leads to light-activated damage. ( b ) AlPcS 2a can be specifically targeted onto lysosomes. Using our staining procedure, AlPcS 2a signals colocalized with Lysotracker Red (top panels) and lamp1-RFP (middle panels), but not with other cellular organelle markers such as EGFP-LC3B (bottom panels, marker for autophagic structures), in HeLa cells. Scale bars, 10 μm. Full size image We first confirmed that selective targeting of AlPcS 2a onto lysosomes can be achieved in our cultured HeLa cell model. Controlled incubation of AlPcS 2a with HeLa cells (Methods) led to the appearance of AlPcS 2a in HeLa cells in the form of small cytoplasmic punctate structures resembling endocytic vesicles. Colocalization experiments with lysosomal markers Lysotracker Red or lamp1-RFP (red fluorescent protein) indicated that AlPcS 2a was indeed recruited selectively onto lysosomes with our labelling scheme ( Fig. 1b ). AlPcS 2a fluorescence, on the other hand, was not found on other organelles, such as peroxisomes, golgi apparatus or mitochondria ( Supplementary Fig. S1 ). AlPcS 2a fluorescence was also absent on autophagic structures, as evident from the lack of colocalization with enhanced green fluorescent protein (EGFP)-LC3B signals ( Fig. 1b ). We next tested the necessary illumination conditions that permit light-mediated lysosomal membrane permeabilization (LMP) in AlPcS 2a -stained HeLa cells. The 635-nm illumination pattern, duration and intensity were finely adjusted to achieve the desired degree of lysosomal damage (see Methods). We found that our optimized light treatment can elicit LMP in a spatiotemporally defined fashion within AlPcS 2a -stained HeLa cells. First, an immediate rise in pH within selected lysosomes could be achieved following light illumination. In HeLa cells co-stained with Lysotracker Red and AlPcS 2a , 635-nm illuminated lysosomes immediately lost their AlPcS 2a fluorescence (due to photobleaching, indicating that the lysosomes were indeed activated by light) as well as their Lysotracker Red signals (due to the rise in pH, Fig. 2a ). Second, our light-illumination conditions led to lysosome impairment without inducing full membrane rupture: fluorescein isothiocyanate (FITC)-dextran (molecular weight=10,000) was retained within light-activated lysosomes in AlPcS 2a -stained HeLa cells ( Fig. 2b ). Furthermore, the retained FITC-dextran fluorescence greatly increased, again confirming that a rise in pH occurred within light-activated lysosomes (FITC pKa=6.5, Fig. 2b ) [19] . With highly selective labelling of AlPcS 2a on the inner membrane of lysosomes, our 635-nm illumination conditions did little damage to other cellular organelles within the same region. Tetramethyl rhodamine ethyl ester perchlorate (TMRE) signals, indicative of active mitochondria (mitochondria are exquisitely sensitive to reactive oxygen species), within the illuminated region remained ( Fig. 2c ). Similarly, luminal markers for ER and peroxisomes were also unaffected upon light activation of lysosomes ( Supplementary Fig. S2 ). This indicated that the methodology could specifically elicit LMP, and was used to further probe the cellular autophagic response following lysosomal damage. Interestingly, we found that trafficking of photo-impaired lysosomes exhibited reduced motility, allowing them to be easily tracked over long periods of time ( Supplementary Fig. S3 ). 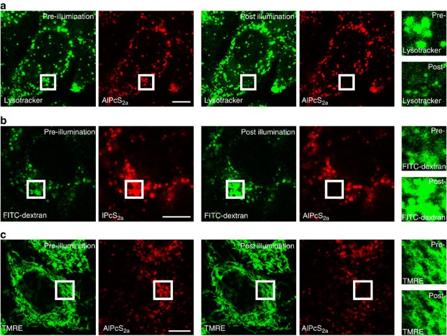Figure 2:Induction ofLMPon individual AlPcS2a-labelled lysosomes. (a) Simultaneous loss of Lysotracker and AlPcS2afluorescence immediately following light activation. A HeLa cell labelled with Lysotracker Red and AlPcS2awas 635-nm illuminated within the white square region (left panels). Lysotracker fluorescence within the illuminated region was immediately lost after light illumination (middle panels), indicating the successful triggering of LMP. Right panels: magnified view of Lysotracker fluorescence within the 635-nm illuminated region pre- and post light activation. (b) 635 nm illumination did not lead to complete lysosome rupture. A HeLa cell labelled with FITC-dextran (molecular weight=10,000) and AlPcS2awas 635-nm illuminated within the white square region (left panels). FITC-dextran remained within illuminated lysosomes (an increase in FITC fluorescence was observed, in accordance with an increase in pH in damaged lysosomes; middle panels). Right panels: magnified view of FITC-dextran fluorescence within the 635-nm illuminated region pre- and post light activation. (c) Light activation did not affect other cellular structures, such as mitochondria. A HeLa cell labelled with TMRE and AlPcS2awas 635-nm illuminated within the white square region (left panels). Illumination did not affect TMRE fluorescence, indicating that mitochondria within the same region were not affected/impaired. Right panels: magnified view of TMRE fluorescence within the 635-nm illuminated region pre- and post light activation. Scale bars, 10 μm. Figure 2: Induction of LMP on individual AlPcS 2a -labelled lysosomes. ( a ) Simultaneous loss of Lysotracker and AlPcS 2a fluorescence immediately following light activation. A HeLa cell labelled with Lysotracker Red and AlPcS 2a was 635-nm illuminated within the white square region (left panels). Lysotracker fluorescence within the illuminated region was immediately lost after light illumination (middle panels), indicating the successful triggering of LMP. Right panels: magnified view of Lysotracker fluorescence within the 635-nm illuminated region pre- and post light activation. ( b ) 635 nm illumination did not lead to complete lysosome rupture. A HeLa cell labelled with FITC-dextran (molecular weight=10,000) and AlPcS 2a was 635-nm illuminated within the white square region (left panels). FITC-dextran remained within illuminated lysosomes (an increase in FITC fluorescence was observed, in accordance with an increase in pH in damaged lysosomes; middle panels). Right panels: magnified view of FITC-dextran fluorescence within the 635-nm illuminated region pre- and post light activation. ( c ) Light activation did not affect other cellular structures, such as mitochondria. A HeLa cell labelled with TMRE and AlPcS 2a was 635-nm illuminated within the white square region (left panels). Illumination did not affect TMRE fluorescence, indicating that mitochondria within the same region were not affected/impaired. Right panels: magnified view of TMRE fluorescence within the 635-nm illuminated region pre- and post light activation. Scale bars, 10 μm. Full size image Damaged lysosomes undergo selective autophagy The hallmark for many forms of selective organelle autophagy is surface ubiquitination. In mitophagy, dysfunctional mitochondria are first ubiquitinated before being turned over [10] , [11] , [13] , [14] , [20] . Artificial ubiquitination of peroxisomal outer-membrane proteins can also lead to pexophagy in mammalian cell cultures [21] , [22] . We therefore probed whether LMP induction through light activation led to selective ubiquitination of impaired (photo-inactivated) lysosomes within a cell region in an EGFP-ubiquitin (EGFP-Ub), lamp1-RFP expressing AlPcS 2a -stained HeLa cell ( Fig. 3a ). Thirty to fifty minutes after illumination, multiple ubiquitin puncta formed within the 635-nm illuminated region ( Fig. 3b ), and these EGFP-Ub fluorescence signals were associated with lamp1-positive, AlPcS 2a -fluorescence-negative puncta ( Fig. 3c ; AlPcS 2a is photobleached in light-impaired lysosomes). On the contrary, active lysosomes that were not illuminated by 635 nm light but were trafficked into the region after illumination were positive for both AlPcS 2a and lamp1, and they did not exhibit strong EGFP-Ub signals, indicating that ubiquitination occurred only on impaired lysosomes. As a control, we quantified three separate regions within the cell for levels of Ub over time, and only the region that has undergone 635 nm illumination (A1, Fig. 3d ) exhibited a time-dependent increase of Ub signal, again highlighting the selectivity of the process. 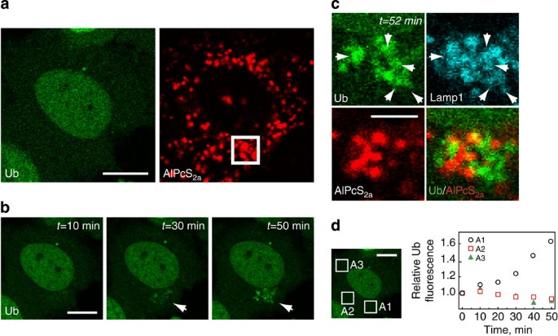Figure 3: Ubiquitination of damaged lysosomes. (a) A HeLa cell expressing EGFP-Ub and lamp1-RFP, and labelled with AlPcS2a, was 635-nm illuminated within the white square region. (b) Punctate structures containing ubiquitin appeared within the 635-nm illuminated region (white arrow) 30–50 min after light activation. (c) Ubiquitin puncta colocalized with damaged lysosomes. Magnified view of the 635-nm illuminated cell region showed that ubiquitin signals localized on lysosomes (lamp1-labelled) lacking AlPcS2afluorescence (indicating that it had been 635-nm illuminated). White arrows indicate examples of Ub on damaged lysosomes. (d) Quantification of ubiquitin signals within three independent cellular regions (A1, A2 and A3) revealed a specific recruitment of ubiquitin to the site of light activation (inset, right, A1). Scale bars, 10 μm (a,b,d); 3 μm (c). Figure 3: Ubiquitination of damaged lysosomes. ( a ) A HeLa cell expressing EGFP-Ub and lamp1-RFP, and labelled with AlPcS 2a , was 635-nm illuminated within the white square region. ( b ) Punctate structures containing ubiquitin appeared within the 635-nm illuminated region (white arrow) 30–50 min after light activation. ( c ) Ubiquitin puncta colocalized with damaged lysosomes. Magnified view of the 635-nm illuminated cell region showed that ubiquitin signals localized on lysosomes (lamp1-labelled) lacking AlPcS 2a fluorescence (indicating that it had been 635-nm illuminated). White arrows indicate examples of Ub on damaged lysosomes. ( d ) Quantification of ubiquitin signals within three independent cellular regions (A1, A2 and A3) revealed a specific recruitment of ubiquitin to the site of light activation (inset, right, A1). Scale bars, 10 μm ( a , b , d ); 3 μm ( c ). Full size image We further monitored whether the specific ubiquitination events observed were indicative of autophagic maintenance on damaged lysosomes. This was first tested in AlPcS 2a -stained HeLa cells expressing TagRFP-p62 and EGFP-Ub ( Fig. 4a ). p62 is a selective autophagy adaptor protein that is recruited onto substrates during selective autophagy, such as in the turnover of dysfunctional mitochondria or protein aggregates [10] , [23] . We observed that spatially restricted induction of ubiquitination as well as p62 accumulation occurred in the light-illuminated region ( Fig. 4b ). p62 and ubiquitin signals were highly associated spatially ( Fig. 4b ), suggesting ubiquitination as a part of the autophagic response against impaired lysosomes. To further this idea, we probed the cell response to light activation in AlPcS 2a -stained HeLa cells expressing EGFP-LC3B and lamp1-RFP ( Fig. 4c ). Lamp1-RFP signals (lysosomes) within the 635-nm illuminated area were initially not colocalized with EGFP-LC3B, but eventually became decorated with the autophagic structure marker LC3, again implicating a selective autophagic action on impaired lysosomes. Western blotting also revealed an accumulation of cellular LC3-II upon global lysosome impairment ( Supplementary Fig. S4a ). This accumulation was much more significant than in Bafilomycin A1 (which blocks the turnover of LC3-II) treated cells, confirming that the observed increase in LC3-II levels within light-illuminated cells mainly reflects an induction of autophagy ( Supplementary Fig. S4b ). Lastly, we demonstrated that our observed autophagic response against lysosome was specific: other forms of selective autophagy, such as parkin-mediated mitophagy, were not induced within the light-illuminated regions ( Supplementary Figs S5 and S6 ). 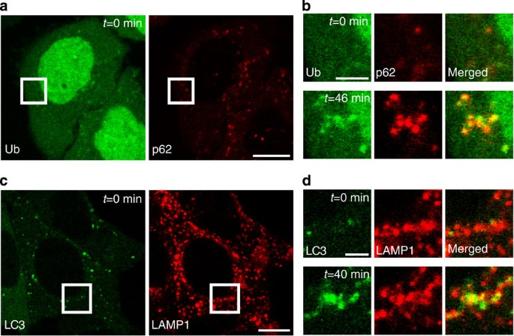Figure 4: Specific recruitment of autophagic adaptor proteins onto damaged lysosomes. (a) A HeLa cell expressing EGFP-Ub and TagRFP-p62, and labelled with AlPcS2a, was 635-nm illuminated within the white square region, resulting in ubiquitination of and p62 recruitment to the photodamaged lysosomes, as shown inb. (b) Magnified view of the 635-nm illuminated cell region ina. Ubiquitin and p62 initially distributed uniformly within the region (t=0 min, top panels), but formed distinct foci after light activation (bottom panels). (c) A HeLa cell expressing EGFP-LC3B and lamp1-RFP, and labelled with AlPcS2a, was 635-nm illuminated within the white square region, resulting in LC3 recruitment onto photodamaged lysosomes, as shown ind. (d) Magnified view of the 635-nm illuminated cell region inc. LC3 is initially distributed away from lysosomes (lamp1,t=0 min, top panels), but appears on lamp1-positive structures 40 min after light activation (bottom panels). Scale bars, 10 μm (a,c); 3 μm (b,d). Figure 4: Specific recruitment of autophagic adaptor proteins onto damaged lysosomes. ( a ) A HeLa cell expressing EGFP-Ub and TagRFP-p62, and labelled with AlPcS 2a , was 635-nm illuminated within the white square region, resulting in ubiquitination of and p62 recruitment to the photodamaged lysosomes, as shown in b . ( b ) Magnified view of the 635-nm illuminated cell region in a . Ubiquitin and p62 initially distributed uniformly within the region ( t =0 min, top panels), but formed distinct foci after light activation (bottom panels). ( c ) A HeLa cell expressing EGFP-LC3B and lamp1-RFP, and labelled with AlPcS 2a , was 635-nm illuminated within the white square region, resulting in LC3 recruitment onto photodamaged lysosomes, as shown in d . ( d ) Magnified view of the 635-nm illuminated cell region in c . LC3 is initially distributed away from lysosomes (lamp1, t =0 min, top panels), but appears on lamp1-positive structures 40 min after light activation (bottom panels). Scale bars, 10 μm ( a , c ); 3 μm ( b , d ). Full size image As only a subset of lysosomes was affected by our method, a cell can maintain normal progression of its autophagic responses (through the remaining healthy lysosome pool). This allowed us to test if the light-damaged lysosomes were successfully turnovered via autophagy using AlPcS 2a -stained HeLa cells expressing RFP-EGFP-LC3 (ref. 24 ). We chose two cells that were undergoing very low levels of basal autophagy for imaging (low amounts of RFP or RFP/EGFP-positive autophagic structures before 635 nm illumination, Fig. 5a ). Local formation of LC3 puncta positive for EGFP fluorescence indicated that autophagic processing of light-impaired lysosomes was activated ( Fig. 5b ). We then tracked whether EGFP fluorescence on these light-induced autophagic structures disappeared over time: EGFP, with a pKa=5.9, loses its fluorescence when autophagosome transition into autolysosomes occurs [24] . Based on this report, we found that the light-induced autophagic structures indeed successfully matured into autolysosomes ( Fig. 5c and Supplementary Fig. S7 ). 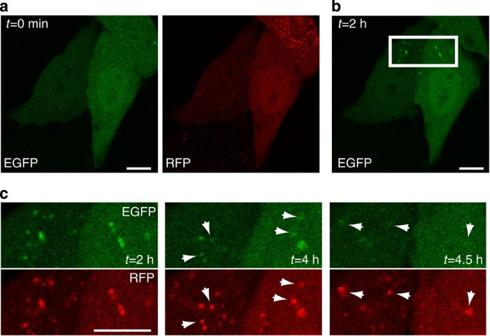Figure 5: Delivery of damaged lysosomes for autophagic turnover. (a) Two HeLa cells expressing RFP-EGFP-LC3 and labelled with AlPcS2awas 635-nm illuminated within the white rectangular region, resulting in local LC3 puncta formation, as shown inb. (b) LC3 puncta were specifically induced within the 635-nm illuminated cell regions ina(LC3 initially distributed uniformly att=0). (c) The loss of EGFP fluorescence from light-induced LC3 puncta preceded the disappearance of RFP fluorescence (white arrows indicate examples of LC3 puncta that exhibited diminished EGFP fluorescence), indicating their successful transition from autophagosomes to autolysosomes. Scale bars, 10 μm. Figure 5: Delivery of damaged lysosomes for autophagic turnover. ( a ) Two HeLa cells expressing RFP-EGFP-LC3 and labelled with AlPcS 2a was 635-nm illuminated within the white rectangular region, resulting in local LC3 puncta formation, as shown in b . ( b ) LC3 puncta were specifically induced within the 635-nm illuminated cell regions in a (LC3 initially distributed uniformly at t =0). ( c ) The loss of EGFP fluorescence from light-induced LC3 puncta preceded the disappearance of RFP fluorescence (white arrows indicate examples of LC3 puncta that exhibited diminished EGFP fluorescence), indicating their successful transition from autophagosomes to autolysosomes. Scale bars, 10 μm. Full size image The findings here add to the role of autophagy in organelle maintenance. Organelles are large cellular structures with complex chemical contents that are perhaps best handled through the autophagic machinery (for example, as compared with the proteasome). Previous reports have shown that damaged mitochondria and peroxisomes can be removed via autophagy. Here we report that photo-impaired lysosomes can also be degraded by similar pathways, and the growing list of organelles that undergo autophagic turnover suggests that autophagy can act as versatile organelle quality-control mechanism in cells. On the other hand, it will be of tremendous interest in the future to pinpoint conditions in which physiologically damaged lysosomes need to undergo autophagic turnover. These efforts will further shed light on the utility of this newly defined pathway. Aside from being as one of the major organelle quality-control mechanisms, the autophagic response towards impaired lysosomes could act as an intrinsic host-defense mechanism against intruding pathogens. Infection is oftentimes established upon breakage of host cell’s vacuolar membranes by pathogens to escape into the cytoplasm [25] . Cellular responses to a break in their vacuolar membrane, such as the autophagic responses reported herein, may allow intruding pathogens to become recaptured for autophagic turnover. Indeed, it has been shown that during Shigella infection, host cell-membrane remnants attached to a bacterium may act as a trigger for autophagy activation [26] . Manipulation of this lysosome-maintenance pathway may therefore represent a useful strategy in combating infectious pathogens. The light-based lysosome-inactivation methodology developed here allowed us to define the lysosome-maintenance pathway within cells. Our methodology represents a robust experimental platform to access the selective lysosomal autophagic process. Questions such as how damaged lysosomes are sensed, as well as what molecular machineries are required for proper lysosome maintenance, can now be dissected. Plasmids EBFP2-parkin was described previously [27] . EBFP2-PMP34 and EGFP2-p62 were constructed through PCR amplification of human genes from HeLa cell total cDNA, followed by its insertion into the EBFP2-Nuc (Addgene plasmid 14893) [28] and EGFP-C1 vectors. EGFP-vkskl plasmid was constructed through appending the DNA sequence encoding amino acids VKSKL to the EGFP-C1 plasmid. The EGFP-Ub, mRFP-GFP-LC3, lamp1-RFP and EGFP-LC3B plasmids were obtained from Addgene (plasmids 11928, 21074, 1817 and 11546) [24] , [29] , [30] , [31] . Cell culture and transfection HeLa cells (ATCC, CCL-2) were cultured in DMEM medium (Life Technologies; 11965), supplemented with 10% FBS (Life Technologies; 10437) and 1% penicillin/streptomycin (Life Technologies; 15140), and maintained at 37 ° C and 5% CO 2 . For transfection into HeLa cells, Lipofectamine 2000 (Life Technologies; 11668) was used based on the manufacturer’s protocol. TMRE (Life Technologies; T-669) was supplemented into cells at 100 nM in cell medium for 20 min at 37 ° C. Mitotracker Green (Life Technologies; M7514) and Lysotracker Red (Life Technologies; L7528) were supplemented into cells at 100 nM in cell medium for 1 h at 37 ° C. BODIPY FL C5-ceramide (Life Technologies; D3521) was supplemented into cells at 5 μM in cell medium for 30 min at 4 ° C, washed two times with PBS and further chased for 30 min at 37 ° C before imaging. EGFP-kdel baculoviruses (Life Technologies; C10590) were used at 20 virus particles per HeLa cell for 24 h. AlPcS 2a labelling A modified AlPcS 2a staining protocol based on previous literature was used [16] . Briefly, a stock solution was prepared by first dissolving 5 mg AlPcS 2a (Frontier Scientific; P40632) in 0.2 ml 0.1 M NaOH, then brought up to a final volume of 1 ml with PBS (final concentration 6.8 mM). This stock solution was filtered through a 0.2-μm filter (Sartorius; 16534) for long-term storage at −20 ° C. To make the staining solution, our AlPcS 2a stock was first diluted to 125 μM in PBS and further diluted 1,000 folds to a final concentration of 125 nM in DMEM. To stain the lysosomes in HeLa cells, the culturing medium was replaced with the staining solution for 16 h at 37 ° C. The cells were then transferred back into the regular culturing medium for an additional 4 h at 37 ° C before imaging. Live-cell manipulation and imaging Light-assisted autophagy was performed on an Olympus FV1000 confocal microscope (60 × , numerical aperture =1.2 water objective or 60 × , numerical aperture =1.3 silicon oil objective) equipped with a SIM scanner. Before observation, the HeLa cells were transferred into phenol red-free medium for observation (Gibco; 31053, containing FBS and P/S). Live HeLa cells were maintained under 37 °C and 5% CO 2 on the microscope for manipulation and observation (Tokai Hit; no. MIU-IBC). To induce LMP with light, we point-scanned a 50-μW 635-nm laser light through a ~7 × 7-μm 2 region in a HeLa cell for a total of 30 s using Olympus FV1000’s tornado scanning. EBFP2 fluorescence was collected using 405 nm excitation (collecting 420–480 nm emission). EGFP fluorescence was collected using 488 nm excitation (collecting 500–550 nm emission), and TagRFP fluorescence was obtained using 559 nm excitation (collecting 575–675 nm emission). AlPcS 2a fluorescence was collected using 635 nm excitation (collecting 655–755 nm emission). A zero-drift compensator module (Olympus) was used to sample drift in the z direction during real-time imaging. The images were not processed after acquisition. Western blotting HeLa cells were scraped into RIPA buffer and centrifuged at 15,000 r.p.m. for 10 min. The supernatant was collected and stored at −20 ° C. Samples were separated by electrophoresis (15% SDS-PAGE), transferred onto polyvinylidene difluoride membranes (Millipore) and probed by anti-LC3B (1:2,000; Novus Biologicals; NB100-2220) and anti-p62 (1:2,000; BD Biosciences; 610832) antibodies. Lysosome motility assay We labelled lysosomes in HeLa cells with Lysotracker Blue (Life Technologies; L7525), FITC-dextran (Life Technologies; D1821) and AlPcS 2a . Intact lysosomes were tracked within single cells through Lysotracker Blue for 30 frames (1.5 s per frame). This was followed by the induction of photodamage on a small fraction of lysosomes through 635 nm illumination (damaged lysosomes showed increased FITC-dextran fluorescence). The photodamaged lysosomes were then tracked for 30 frames (1.5 s per frame) through FITC-dextran fluorescence. Individual lysosome trajectories were analysed through the particle tracker plugin in Image J. RFP-GFP-LC3 analysis GFP/RFP intensity ratios at different time points were analysed by MATLAB. Images were thresholded for autophagic structure identification and calculated for GFP/RFP intensity ratios over time. How to cite this article: Hung, Y.-H. et al. Spatiotemporally controlled induction of autophagy-mediated lysosome turnover. Nat. Commun. 4:2111 doi: 10.1038/ncomms3111 (2013).